Control of synaptic vesicle endocytosis by an extracellular signalling molecule Signalling cascades control multiple aspects of presynaptic function. Synaptic vesicle endocytosis was assumed to be exempt from modulation, due to its essential role maintaining synaptic vesicle supply and thus neurotransmission. Here we show that brain-derived neurotrophic factor arrests the rephosphorylation of the endocytosis enzyme dynamin I via an inhibition of glycogen synthase kinase 3. This event results in a selective inhibition of activity-dependent bulk endocytosis during high-intensity firing. Furthermore, the continued presence of brain-derived neurotrophic factor alleviates the rundown of neurotransmission during high activity. Thus, synaptic strength can be modulated by extracellular signalling molecules via a direct inhibition of a synaptic vesicle endocytosis mode. Neurotransmitter release from central nerve terminals is modulated by multiple signalling cascades activated by extracellular ligands [1] . This process facilitates the fine control of synaptic output by either inhibitory/excitatory neurotransmission or retrograde neurotransmitters. In contrast synaptic vesicle (SV) endocytosis has not been demonstrated to be modulated by extracellular signalling cascades, presumably due to its obligatory role in maintaining the available stock of SVs inside nerve terminals. SVs are retrieved from the nerve terminal plasma membrane after exocytosis by either clathrin-mediated endocytosis (CME) or activity-dependent bulk endocytosis (ADBE). CME is the dominant SV retrieval mode during low intensity stimulation [2] , [3] and retrieves single SVs de novo from the plasma membrane. In contrast, ADBE is triggered during high-intensity stimulation and forms endosomes directly from large plasma membrane invaginations [4] . SVs then bud from these endosomes in a clathrin- and adaptor protein-dependent manner [5] , [6] , [7] . ADBE is tightly coupled to neuronal activity via the dephosphorylation of the large GTPase dynamin I at two sites (Ser-774 and Ser-778) by the calcium-dependent phosphatase calcineurin [8] . After stimulation terminates dynamin I is rephosphorylated firstly on Ser-778 by the constitutively active enzyme cyclin-dependent kinase 5 (cdk5), an event which permits phosphorylation of Ser-774 by glycogen synthase kinase 3 (GSK3) [9] . The rephosphorylation of dynamin I by either cdk5 or GSK3 is essential for the triggering of ADBE by subsequent stimuli [9] , [10] . Brain-derived neurotrophic factor (BDNF) has established roles in the long-term control of neuronal migration, survival and development [11] . In addition to its trophic actions, acute exposure to BDNF has both presynaptic and postsynaptic effects on neurotransmission [11] , [12] . BDNF signals through the TrkB receptor to activate a number of intracellular signalling cascades, such as the mitogen-activated protein kinase (MAPK), the phospholipase Cγ and phosphatidylinositol 3-kinase (PI3K) pathways. Activation of the PI3K pathway results in a downstream inhibition of GSK3 (ref. 13) ; therefore, we hypothesized that BDNF may negatively control ADBE via an inhibition of dynamin I rephosphorylation. We show that application of BDNF inhibits GSK3-dependent rephosphorylation of Ser-774 on dynamin I via a PI3K cascade. Furthermore, we find that BDNF negatively regulates ADBE, and that this inhibition results in an enhancement of neurotransmission but only after a prior priming stimulus. Thus, we have shown that extracellular signalling molecules can modulate neurotransmission via a differential control of a key SV endocytosis mode. BDNF inhibits dynamin I rephosphorylation on Ser-774 The rephosphorylation of Ser-774 on dynamin I by GSK3 is essential for the triggering of multiple cycles of ADBE [9] . This suggests that ADBE should be negatively regulated by signalling cascades that inhibit GSK3 activity, as blocking dynamin I rephosphorylation arrests this endocytosis mode. One potential signalling molecule that could inhibit ADBE is BDNF, as it can inhibit GSK3 via activation of a PI3K-dependent cascade [12] ( Fig. 1a ). To test this hypothesis, we first confirmed that BDNF could control GSK3 activity in our primary neuronal culture system, cerebellar granule neurons (CGNs). GSK3 activity can be reported by the extent of phosphorylation of Ser-9 on the enzyme using phosphorylation-specific antibodies. In CGNs, Akt is activated by high-frequency stimulation and transiently phosphorylates GSK3 on Ser-9 (ref. 14 ). This effect was replicated in this study, with strong stimulation evoking a transient phosphorylation of both Akt and GSK3 which returned to resting levels on repolarization of the cultures ( Fig. 1c,e ). Application of BDNF (100 ng ml −1 ) resulted in a hyperphosphorylation of both Akt and GSK3 in all experimental conditions ( Fig. 1c,e ), indicating BDNF triggers an intracellular signalling cascade that phosphorylates both Akt and GSK3. 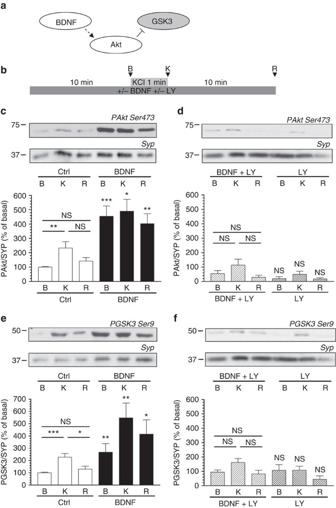Figure 1: BDNF inhibits GSK3 activity via a PI3K-dependent cascade. (a) Scheme illustrating that BDNF would activate a signalling cascade, which would phosphorylate and inactivate GSK3. (b) CGNs were placed in incubation medium for 10 min before stimulation with 50 mM KCl (1 min). Following stimulation CGNs were repolarized for 10 min. Samples were prepared from cultures before stimulation (basal, B), directly after KCl stimulation (K) or after 10 min repolarization (R) as indicated by arrowheads. BDNF (100 ng ml−1) or LY294002 (LY, 10 μM) were present throughout the experiment where indicated. Lysates were separated by SDS–PAGE and probed for either (c,d) phospho-Ser-473 on Akt (PAkt Ser473) or (e,f) phospho-Ser-9 on GSK3 (PGSK3 Ser-9) on immunoblots. Quantitative analysis is shown in the graphs in (c–f). These graphs display the extent of phosphorylation of either Ser-473 on Akt (c,d) or Ser-9 on GSK3 (e,f). All values were normalized to the amount of synaptophysin (SYP) as a loading control, and expressed as a percentage of Basal control±s.e.m. (c)n=7, (d)n=6, (e)n=7, (f)n=6; one-way ANOVA. *P<0.05, **P<0.01, ***P<0.001 compared with basal control unless indicated. Figure 1: BDNF inhibits GSK3 activity via a PI3K-dependent cascade. ( a ) Scheme illustrating that BDNF would activate a signalling cascade, which would phosphorylate and inactivate GSK3. ( b ) CGNs were placed in incubation medium for 10 min before stimulation with 50 mM KCl (1 min). Following stimulation CGNs were repolarized for 10 min. Samples were prepared from cultures before stimulation (basal, B), directly after KCl stimulation (K) or after 10 min repolarization (R) as indicated by arrowheads. BDNF (100 ng ml −1 ) or LY294002 (LY, 10 μM) were present throughout the experiment where indicated. Lysates were separated by SDS–PAGE and probed for either ( c , d ) phospho-Ser-473 on Akt ( PAkt Ser473 ) or ( e , f ) phospho-Ser-9 on GSK3 ( PGSK3 Ser-9 ) on immunoblots. Quantitative analysis is shown in the graphs in ( c – f ). These graphs display the extent of phosphorylation of either Ser-473 on Akt ( c , d ) or Ser-9 on GSK3 ( e , f ). All values were normalized to the amount of synaptophysin (SYP) as a loading control, and expressed as a percentage of Basal control ± s.e.m. ( c ) n =7, ( d ) n =6, ( e ) n =7, ( f ) n =6; one-way ANOVA. * P <0.05, ** P <0.01, *** P <0.001 compared with basal control unless indicated. Full size image We next determined which intracellular signalling cascade BDNF was operating through to control GSK3 activity. We first investigated the potential role of TrkB receptors as they are highly expressed in CGNs [15] , [16] . Application of the tyrosine kinase antagonist K252a inhibited BDNF-induced phosphorylation of both Akt and GSK3, indicating a TrkB-specific effect ( Supplementary Fig. S1 ). TrkB receptors signal via multiple intracellular signalling cascades, one of which utilizes PI3K [12] . In this cascade production of PI(3,4,5)P 3 by PI3K activates phosphoinositide-dependent kinase 1 (PDK1) to phosphorylate and activate Akt. To determine whether BDNF signals via PI3K, the selective antagonist LY294002 (10 μM) was applied to CGNs. LY294002 abolished BDNF-induced hyperphosphorylation of both Akt and GSK3 ( Fig. 1d,f ) indicating BDNF exerts its effect via a PI3K-dependent cascade. Phosphorylation of GSK3 inhibits its activity, therefore we next assessed whether BDNF could control dynamin I Ser-774 rephosphorylation, an event mediated by this enzyme [9] ( Fig. 2a ). In the absence of BDNF, Ser-774 was dephosphorylated on depolarization, and then rephosphorylated on removal of the stimulus ( Fig. 2c ). This rephosphorylation event was abolished in the presence of BDNF ( Fig. 2c ). Importantly, BDNF had no effect on the rephosphorylation of Ser-778 on dynamin I ( Fig. 2e ), an event mediated by cdk5 (ref. 9 ). Thus, BDNF selectively inhibits the rephosphorylation of Ser-774 on dynamin I via inhibition of GSK3. 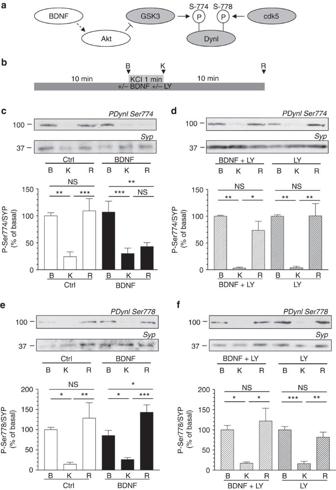Figure 2: BDNF inhibits dynamin I rephosphorylation on Ser-774 via a PI3K-dependent cascade. (a) Scheme illustrating that cdk5 phosphorylates Ser-778 on dynamin I (DynI), allowing GSK3 to phosphorylate Ser-774. Our hypothesis was that BDNF would activate Akt to phosphorylate and inactivate GSK3, thus inhibiting its ability to rephosphorylate Ser-774 on DynI. (b) CGNs were placed in incubation medium for 10 min before stimulation with 50 mM KCl (1 min). Following stimulation, CGNs were repolarized for 10 min. Samples were prepared from cultures before stimulation (basal, B), directly after KCl stimulation (K) or after 10 min repolarization (R) as indicated by arrowheads. BDNF (100 ng ml−1) or LY294002 (LY, 10 μM) were present throughout the experiment where indicated. Lysates were separated by SDS–PAGE and probed for either (c,d) phospho-Ser-774 (PDynI Ser-774) or (e,f) phospho-Ser-778 (PDynI Ser-778) on dynamin I on immunoblots. Quantitative analysis is shown in the graphs in (c–f). These graphs display the extent of phosphorylation of either Ser-774 (c,d) or Ser-778 (e,f). All values were normalized to the amount of synaptophysin (SYP) as a loading control, and expressed as a percentage of Basal±s.e.m. (c)n=9, (d)n=3, (e)n=5, (f)n=4, one-way analysis of variance (ANOVA). *P<0.05, **P<0.01, ***P<0.001. Figure 2: BDNF inhibits dynamin I rephosphorylation on Ser-774 via a PI3K-dependent cascade. ( a ) Scheme illustrating that cdk5 phosphorylates Ser-778 on dynamin I (DynI), allowing GSK3 to phosphorylate Ser-774. Our hypothesis was that BDNF would activate Akt to phosphorylate and inactivate GSK3, thus inhibiting its ability to rephosphorylate Ser-774 on DynI. ( b ) CGNs were placed in incubation medium for 10 min before stimulation with 50 mM KCl (1 min). Following stimulation, CGNs were repolarized for 10 min. Samples were prepared from cultures before stimulation (basal, B), directly after KCl stimulation (K) or after 10 min repolarization (R) as indicated by arrowheads. BDNF (100 ng ml −1 ) or LY294002 (LY, 10 μM) were present throughout the experiment where indicated. Lysates were separated by SDS–PAGE and probed for either ( c , d ) phospho-Ser-774 ( PDynI Ser-774 ) or ( e , f ) phospho-Ser-778 ( PDynI Ser-778 ) on dynamin I on immunoblots. Quantitative analysis is shown in the graphs in ( c – f ). These graphs display the extent of phosphorylation of either Ser-774 ( c , d ) or Ser-778 ( e , f ). All values were normalized to the amount of synaptophysin (SYP) as a loading control, and expressed as a percentage of Basal ± s.e.m. ( c ) n =9, ( d ) n =3, ( e ) n =5, ( f ) n =4, one-way analysis of variance (ANOVA). * P <0.05, ** P <0.01, *** P <0.001. Full size image We next examined whether inhibition of PI3K could reverse the observed effects of BDNF on GSK3-dependent dynamin I Ser-774 rephosphorylation. This was the case, with application of LY294002 preventing the BDNF-mediated inhibition of dynamin I Ser-774 rephosphorylation ( Fig. 2d ), while having no effect on cdk5-dependnet Ser-778 rephosphorylation ( Fig. 2f ). Thus, GSK3-dependent phosphorylation of Ser-774 is negativity regulated by a PI3K/PDK1/Akt signalling cascade that is triggered by BDNF. BDNF selectively inhibits ADBE GSK3-dependent Ser-774 rephosphorylation controls ADBE [9] , therefore inhibition of this event by BDNF has implications for presynaptic function during elevated neuronal activity. Therefore, we next determined whether BDNF could negatively control ADBE. First, we examined the uptake of large (40 kDa) fluorescent dextrans, as they specifically report fluid phase uptake via ADBE due to size exclusion from SVs [4] , [9] . Acute application of BDNF had no effect on dextran uptake evoked by a train of high-frequency action potentials (80 Hz, 10 s, Fig. 3a ). However, inhibition of dynamin I Ser-774 rephosphorylation will not be apparent under these conditions, as dynamin I is highly phosphorylated at rest and dephosphorylated on stimulation ( Fig. 2c ). To reveal a potential regulatory effect of BDNF on ADBE, cultures were challenged with a priming stimulus to dephosphorylate dynamin I, rested in the continued presence of BDNF (to inhibit dynamin I rephosphorylation) and then dextran uptake was assessed during a second stimulation ( Fig. 3b ). Under these conditions, BDNF produced a robust inhibition of dextran uptake, which was prevented by the PI3K antagonist LY294002 ( Fig. 3b ). This inhibition was occluded by the GSK3 antagonist CT99021 ( Fig. 3b ) indicating BDNF was mediating its effect via this enzyme and almost certainly via inhibition of Ser-774 rephosphorylation. A BDNF-dependent inhibition of ADBE was also observed in primary hippocampal cultures, indicating its effect was not limited to cerebellar neurons ( Supplementary Fig. S2 ). 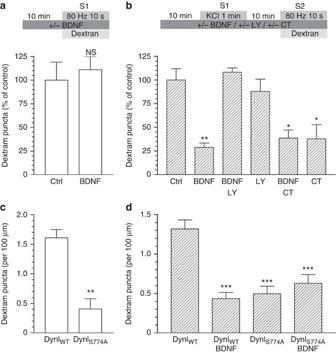Figure 3: BDNF inhibition of protein rephosphorylation by GSK3 arrests dextran uptake. (a) CGNs or (c) CGNs transfected with either wild-type (DynIWT) or S774A dynamin I mutant (DynIS774A) were placed in incubation medium for 10 min before stimulation with a train of 800 action potentials (80 Hz) in the presence of 50 μM tetramethylrhodamine dextran. (b) CGNs or (d) CGNs transfected with either wild-type (DynIWT) or S774A dynamin I mutant (DynIS774A) were placed in incubation medium for 10 min before a priming stimulus of 50 mM KCl (1 min). CGNs were then repolarized for 10 min before stimulation with 800 action potentials (80 Hz) in the presence of 50 μM tetramethylrhodamine dextran. BDNF (100 ng ml−1), LY294002 (LY, 10 μM) or CT99021 (CT, 2 μM) were present throughout the experiment where indicated. Dextran was perfused away immediately after stimulation in both cases. (a,b) The number of dextran puncta expressed as a percentage of control corrected for the unstimulated background±s.e.m., (a) Ctrl and BDNFn=5; Student’st-testP=0.69, (b) Ctrln=10, BDNFn=4, BDNF/LYn=4, LYn=7, BDNF/CTn=3, CTn=3 one-way analysis of variance (ANOVA). *P<0.05, **P<0.01 compared with control. (c,d) The average number of dextran puncta per 100 μm of transfected neuron corrected for unstimulated background±s.e.m., (c) bothn=3; Student’st-testP=0.006, (d) DynIWTn=5, all othersn=3, one-way ANOVA. ***P<0.001 compared with DynIWT. Figure 3: BDNF inhibition of protein rephosphorylation by GSK3 arrests dextran uptake. ( a ) CGNs or ( c ) CGNs transfected with either wild-type (DynI WT ) or S774A dynamin I mutant (DynI S774A ) were placed in incubation medium for 10 min before stimulation with a train of 800 action potentials (80 Hz) in the presence of 50 μM tetramethylrhodamine dextran. ( b ) CGNs or ( d ) CGNs transfected with either wild-type (DynI WT ) or S774A dynamin I mutant (DynI S774A ) were placed in incubation medium for 10 min before a priming stimulus of 50 mM KCl (1 min). CGNs were then repolarized for 10 min before stimulation with 800 action potentials (80 Hz) in the presence of 50 μM tetramethylrhodamine dextran. BDNF (100 ng ml −1 ), LY294002 (LY, 10 μM) or CT99021 (CT, 2 μM) were present throughout the experiment where indicated. Dextran was perfused away immediately after stimulation in both cases. ( a , b ) The number of dextran puncta expressed as a percentage of control corrected for the unstimulated background ± s.e.m., ( a ) Ctrl and BDNF n =5; Student’s t -test P =0.69, ( b ) Ctrl n =10, BDNF n =4, BDNF/LY n =4, LY n =7, BDNF/CT n =3, CT n =3 one-way analysis of variance (ANOVA). * P <0.05, ** P <0.01 compared with control. ( c , d ) The average number of dextran puncta per 100 μm of transfected neuron corrected for unstimulated background ± s.e.m., ( c ) both n =3; Student’s t -test P =0.006, ( d ) DynI WT n =5, all others n =3, one-way ANOVA. *** P <0.001 compared with DynI WT . Full size image To confirm that Ser-774 on dynamin I was the principal target of BDNF, we repeated the dextran uptake experiments in neurons expressing either wild-type dynamin I or a phospho-null version mutated at Ser-774. Neurons expressing the S774A mutant displayed a large inhibition of dextran uptake at S1 compared with wild-type, as previously shown [9] ( Fig. 3c ). The S774A mutant inhibited dextran uptake at S2 to an almost identical extent, with the level of inhibition equal to wild-type expressing neurons in the presence of BDNF ( Fig. 3d ). Importantly, BDNF did not reduce dextran uptake further in S774A-expressing neurons ( Fig. 3d ) providing compelling evidence that BDNF inhibits ADBE via arrest of dynamin I Ser-774 phosphorylation, but only after a prior priming stimulus. To confirm the negative control of ADBE by BDNF, morphological studies were performed examining uptake of the fluid phase marker horse radish peroxidase (HRP). Triggering of ADBE results in the appearance of HRP-labelled endosomes, whereas CME generates HRP-labelled SVs [4] ( Fig. 4b–e ). Acute application of BDNF had no effect on the number of HRP-labelled endosomes generated by a strong stimulation ( Fig. 4f ). However, when BDNF was present during and after a priming depolarization (S1) the number of HRP-labelled endosomes generated by a second stimulus (S2) was significantly reduced ( Fig. 4f ). Importantly, BDNF had no effect on the number of HRP-labelled SVs at either S1 or S2 ( Fig. 4g ), indicating no effect on CME. Thus, using two independent assays, BDNF negatively controls ADBE when present during a prior priming stimulus. 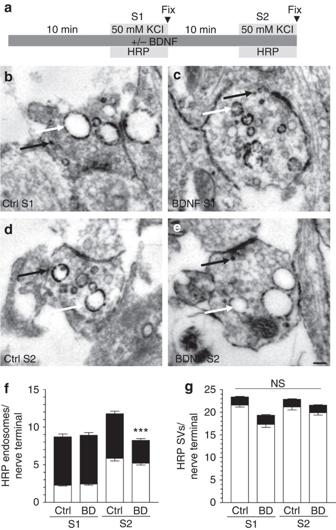Figure 4: BDNF arrests HRP-endosome formation after prior stimulation. (a) CGNs were placed in incubation medium for 10 min before stimulation with 50 mM KCl for 2 min (S1). CGNs were then repolarized for 10 min before a second stimulus with 50 mM KCl (S2). HRP (10 mg ml−1) was co-applied with KCl at either S1 or S2 and CGNs were immediately fixed after stimulation as indicated by arrowheads. BDNF (100 ng ml−1) was present the throughout experiment where indicated. Representative images display typical nerve terminals at S1 for either Ctrl (b) or BDNF (c) and at S2 for either Ctrl (d) or BDNF (e). White arrows indicate HRP-labelled endosomes, black arrows indicate HRP-labelled SVs. Scale bar, 150 nm forb–e. Mean number of HRP-labelled (solid bars) or empty (open bars) endosomes (f) or SVs (g) at either S1 or S2 in control (Ctrl) or BDNF-treated (BD) cells±s.e.m. (n=3 independent experiments for all conditions; one-way analysis of variance (ANOVA). ***P<0.001 compared with all other conditions). Figure 4: BDNF arrests HRP-endosome formation after prior stimulation. ( a ) CGNs were placed in incubation medium for 10 min before stimulation with 50 mM KCl for 2 min (S1). CGNs were then repolarized for 10 min before a second stimulus with 50 mM KCl (S2). HRP (10 mg ml −1 ) was co-applied with KCl at either S1 or S2 and CGNs were immediately fixed after stimulation as indicated by arrowheads. BDNF (100 ng ml −1 ) was present the throughout experiment where indicated. Representative images display typical nerve terminals at S1 for either Ctrl ( b ) or BDNF ( c ) and at S2 for either Ctrl ( d ) or BDNF ( e ). White arrows indicate HRP-labelled endosomes, black arrows indicate HRP-labelled SVs. Scale bar, 150 nm for b – e . Mean number of HRP-labelled (solid bars) or empty (open bars) endosomes ( f ) or SVs ( g ) at either S1 or S2 in control (Ctrl) or BDNF-treated (BD) cells ± s.e.m. ( n =3 independent experiments for all conditions; one-way analysis of variance (ANOVA). *** P <0.001 compared with all other conditions). Full size image BDNF increases both evoked and spontaneous neurotransmitter release in a number of experimental systems [12] . To determine whether this occurred in our culture system we monitored SV-fusion events using the pH-sensitive genetic reporter sypHy [2] . SypHy is the SV protein synaptophysin with a-pH-sensitive GFP fused to one of its luminal loops. It reports SV exocytosis as its fluorescence is quenched by the acidic interior of the SV, and then unquenched as the SV fuses and encounters the neutral pH of the extracellular medium. To isolate SV exocytosis from subsequent SV endocytosis and reacidification, we inhibited the vesicular ATPase with bafilomycin A1. During 10 min of bafilomycin A1 treatment, the sypHy response gradually increased in transfected neurons, indicative of spontaneous SV fusion [17] ( Fig. 5a ). BDNF was co-applied with bafilomycin A1 to determine whether it would increase spontaneous activity ( Fig. 5a ). No significant difference in sypHy fluorescence was observed during the 10 min incubation period compared with control ( Fig. 5 ), suggesting that BDNF did not alter spontaneous SV turnover in our cultures. After 10 min, a train of 800 action potentials (80 Hz) was delivered to evoke SV fusion in either BDNF-treated or control neurons. A robust increase in sypHy fluorescence was observed in both conditions, which was unaffected by the presence of BDNF ( Fig. 5a,b ), indicating no effect on evoked SV fusion. To confirm a lack of effect of BDNF on SV exocytosis in our culture system, we monitored the extent of unloading of the fluorescent dye FM2-10 after application of BDNF. Exposure to BDNF elicited no change in the extent of SV fusion when compared with control neurons ( Supplementary Fig. S3 ). Therefore, BDNF selectively inhibits ADBE during high-frequency stimulation in CGN nerve terminals. 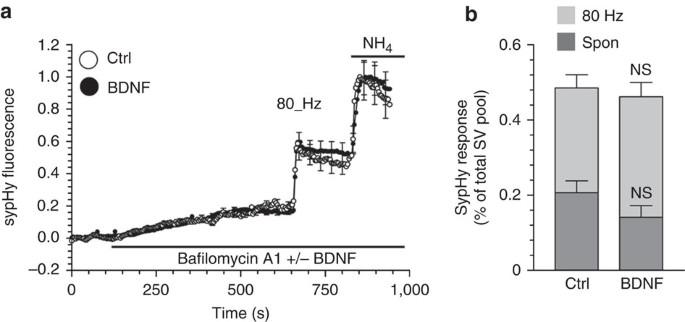Figure 5: BDNF has no effect on SV exocytosis. CGNs expressing sypHy were placed in incubation medium for 10 min. The sypHy fluorescence response was then monitored for 40 s before addition of bafilomycin A1 (200 nM). After 10 min, CGNs were stimulated with a train of 800 action potentials (80 Hz). Finally, cultures were exposed to 50 mM NH4Cl. (a) Representative traces of the sypHy response in the presence (solid) or absence (clear, Ctrl) of BDNF (100 ng ml−1) are displayed showing the response to bafilomycin A1, action potentials and NH4Cl (indicated by bars). Traces are normalized to the NH4Cl pulse. (b) Quantified data showing the extent of spontaneous (Spon, dark grey) and evoked (80 Hz, light grey) SV exocytosis in the absence (Ctrl) or presence (BDNF) of BDNF. Both values are displayed as a proportion of the total SV pool±s.e.m., Ctrl,n=4, BDNF,n=5 independent experiments, Student’st-testP=0.17 for spontaneous andP=0.45 for evoked. Figure 5: BDNF has no effect on SV exocytosis. CGNs expressing sypHy were placed in incubation medium for 10 min. The sypHy fluorescence response was then monitored for 40 s before addition of bafilomycin A1 (200 nM). After 10 min, CGNs were stimulated with a train of 800 action potentials (80 Hz). Finally, cultures were exposed to 50 mM NH 4 Cl. ( a ) Representative traces of the sypHy response in the presence (solid) or absence (clear, Ctrl) of BDNF (100 ng ml −1 ) are displayed showing the response to bafilomycin A1, action potentials and NH 4 Cl (indicated by bars). Traces are normalized to the NH 4 Cl pulse. ( b ) Quantified data showing the extent of spontaneous (Spon, dark grey) and evoked (80 Hz, light grey) SV exocytosis in the absence (Ctrl) or presence (BDNF) of BDNF. Both values are displayed as a proportion of the total SV pool ± s.e.m., Ctrl, n =4, BDNF, n =5 independent experiments, Student’s t -test P =0.17 for spontaneous and P =0.45 for evoked. Full size image BDNF sustains neurotransmission during high-frequency stimuli The selective control of ADBE by BDNF suggests that it should modulate neurotransmission during high-frequency firing, as ADBE is the dominant mechanism of SV retrieval under these conditions [4] . To test this, we examined the effect of applying BDNF on neurotransmission at the parallel fibre—Purkinje cell synapse in intact cerebellar slices. Specifically, we determined the effect of BDNF on synaptic depression, where neurotransmission is progressively decreased during a high-frequency train of action potentials. This depression is exacerbated when CME is inhibited, reflecting a depletion of available SVs for release [18] , [19] , [20] . Application of BDNF had no effect on the evoked depression in slices (600 action potentials, 40 Hz) when it was added 1 h before stimulation ( Supplementary Fig. S4 ). In contrast, slices that had experienced a prior identical depolarizing stimulus in the presence of BDNF exhibited a profound relief of depression when challenged with a second stimulus (S2) 10 min later ( Fig. 6a,b ). This relief of depression at S2 was prevented by the presence of LY294002 and occluded by CT99021 ( Fig. 6c–f ), indicating that this effect was mediated by the same cascade that controls GSK3 rephosphorylation of Ser-774 on dynamin I. The relief of depression was not due to an increase in release probability, as paired pulse facilitation was not altered at either S1 or S2 by BDNF ( Supplementary Fig. S5 ). Thus, BDNF enhances synaptic transmission during high-intensity firing via a negative control of both GSK3 activity and ADBE. 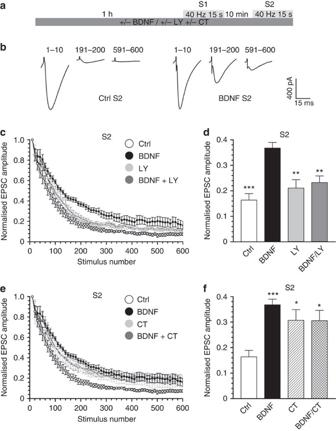Figure 6: BDNF relieves synaptic depression at cerebellar synapses. (a) Cerebellar slices were incubated with combinations of either BDNF (100 ng ml−1), LY294002 (LY 10 μM) or CT99021 (2 μM) for 1 h before being transferred to the recording chamber. Slices were challenged with 600 action potentials (40 Hz, S1) then allowed to recover for 10 min before a second challenge with an identical stimulus train. (b) Example mean EPSCs recorded at three time points during the train of 600 stimuli. The numbers above denote the sweep numbers that were averaged to obtain the trace. (c,e) Summary plots showing the dependence of the EPSC amplitude on the stimulus number at S2. The first EPSC was normalized to 1 to allow direct comparison of the different recording conditions on the rundown of the amplitudes of the EPSCs. (d,f) The mean EPSC amplitude after 200 action potentials is displayed for each experimental condition±s.e.m. (Ctrln=11, BDNFn=9, LYn=7, BDNF/LYn=9, CTn=9, BDNF/CTn=9; one-way analysis of variance (ANOVA) in (e). ***P<0.001, **P<0.01 compared with BDNF; in (f) ***P<0.001, *P<0.05 compared with Ctrl; all other conditions were not significant to each other). Figure 6: BDNF relieves synaptic depression at cerebellar synapses. ( a ) Cerebellar slices were incubated with combinations of either BDNF (100 ng ml −1 ), LY294002 (LY 10 μM) or CT99021 (2 μM) for 1 h before being transferred to the recording chamber. Slices were challenged with 600 action potentials (40 Hz, S1) then allowed to recover for 10 min before a second challenge with an identical stimulus train. ( b ) Example mean EPSCs recorded at three time points during the train of 600 stimuli. The numbers above denote the sweep numbers that were averaged to obtain the trace. ( c , e ) Summary plots showing the dependence of the EPSC amplitude on the stimulus number at S2. The first EPSC was normalized to 1 to allow direct comparison of the different recording conditions on the rundown of the amplitudes of the EPSCs. ( d , f ) The mean EPSC amplitude after 200 action potentials is displayed for each experimental condition ± s.e.m. (Ctrl n =11, BDNF n =9, LY n =7, BDNF/LY n =9, CT n =9, BDNF/CT n =9; one-way analysis of variance (ANOVA) in ( e ). *** P <0.001, ** P <0.01 compared with BDNF; in ( f ) *** P <0.001, * P <0.05 compared with Ctrl; all other conditions were not significant to each other). Full size image Presynaptic control of neurotransmitter release is a well-established phenomenon and involves control of the SV-fusion event via modulation of either neuronal excitability, calcium influx or release probability [21] . We have shown that extracellular signalling molecules can also control SV endocytosis during high-intensity stimulation, with subsequent consequences for neurotransmission. This work reveals a novel regulatory mechanism to control neurotransmission during high-intensity stimulation and to our knowledge this is the first demonstration of an extracellular signalling cascade controlling SV endocytosis. Where possible we evoked ADBE using high-frequency action potentials, however, the design of particular experiments necessitated the use of elevated KCl. We have extensively characterized these two stimuli in our culture system and have found that in terms of (1) the extent of SV exocytosis evoked [22] , (2) the amount of ADBE and CME triggered [23] , (3) the replenishment of both the RRP and reserve pools [24] and (4) the extent of Akt and GSK3 phosphorylation [14] , application of 50 mM KCl is equivalent to the delivery of 800 action potentials at 80 Hz. GSK3-dependent phosphorylation of Ser-774 on dynamin I is essential for ADBE to proceed [9] . As GSK3 activity is negatively regulated by phosphorylation, we searched for potential candidate signalling molecules that may control ADBE. BDNF was selected for study as CGNs express TrkB receptors [15] , [16] and BDNF is released in an activity-dependent manner from central neurons [25] , [26] , [27] , [28] . We show that BDNF mediates its action via a PI3K-dependent intracellular signalling cascade that activates Akt to inhibit GSK3, resulting in arrest of dynamin Ser-774 rephosphorylation. We could not directly test the effect of TrkB receptor inhibition on dynamin I rephosphorylation, as K252a reduced Ser-774 rephosphorylation by ~80% in the absence of BDNF. A key point relating to the inhibition of dynamin I rephosphorylation via this cascade is that the effects of BDNF on both ADBE and neurotransmission are only revealed after a priming stimulus. Thus, there is no acute effect of this cascade on either process, providing compelling evidence that the mechanism by which BDNF acts is a protein rephosphorylation event that occurs after stimulation terminates. In agreement, identical results on ADBE and neurotransmission were observed using either cdk5 or GSK3 antagonists [9] , [10] . BDNF increases spontaneous and evoked neurotransmitter release in a number of neuronal systems [29] , [30] , [31] , [32] , [33] , [34] . However, other studies have reported no effect on baseline transmission [30] , [35] , [36] , [37] . The presynaptic mechanism by which BDNF increases glutamate release is TrkB-dependent [38] and mediated by an intracellular MAPK-signalling cascade [34] . Phosphorylation of the SV protein synapsin is essential in mediating the BDNF effect, as either synapsin I knockout or mutation of the MAPK phosphorylation site on synapsin I negated this effect [34] , [39] . A requirement for the myosin VI motor complex has also been proposed, potentially involving an actin-dependent delivery of SVs [40] . In our culture system, we see no enhancement of evoked SV exocytosis by BDNF. This is most probably due to the stimulation conditions, which were specifically chosen to ensure any facilitation of SV exocytosis by BDNF would be minimal. Thus, by evoking near maximal responses (required to trigger ADBE) we have also allowed the BDNF-dependent modulation of SV endocytosis to be isolated from potentially complicating facilitatory effects on SV exocytosis. We observed a robust relief of synaptic depression by BDNF at cerebellar synapses, which was only revealed after a prior train of action potentials. Previous work in hippocampal neurons has shown that BDNF increases post-tetanic potentiation, via a MAPK-dependent phosphorylation of synapsin I [39] . To eliminate a potential complication due to this effect, conditions were established to discount any increase in quantal content by normalizing all EPSCs to the first pulse. Furthermore, we see a complete reversal of BDNF effects by inhibition of PI3K, eliminating a potential role for MAPK. Finally, we see no effects on release probability by application of BDNF in our cerebellar slice system, in agreement with previous observations which showed minimal effects on paired pulse facilitation on BDNF application [41] . BDNF has both presynaptic and postsynaptic [42] effects, therefore to ensure any modulation of GSK3 was presynaptic, we included the GSK3 antagonist CT99021 in the patch pipette. The fact that no effect was observed on neurotransmission during the first train of high-frequency stimulation also ruled out other postsynaptic intracellular signalling cascades from playing a BDNF-dependent role. Thus, the relief of synaptic depression by BDNF only after a prior stimulation strongly indicates a presynaptic role for BDNF. The relief of synaptic depression by BDNF agrees with studies in hippocampal slices, which showed that inhibition of either presynaptic GSK3 or knockout of syndapin I (both of which arrest ADBE) resulted in a relief of neurotransmission [9] , [43] . Thus, agents that block ADBE seem to increase synaptic transmission in contrast to inhibition of CME, which exacerbates a depression [18] , [19] , [20] . The mechanism by which this occurs is still unclear. For example, there is no consistent increase in either the extent of CME [9] , [10] , [23] or RRP size [24] during inhibition of ADBE in neuronal culture. Another possibility is that SV turnover is more efficient when ADBE is inhibited, as all available SV membrane and cargo will be packaged into release ready SVs at the plasma membrane, rather than via a series of endosomal intermediates [7] . Regardless of mechanism, it is becoming apparent that modulation of SV endocytosis modes could be a route for bidirectional manipulation of neurotransmission during high-frequency firing. A key question raised by this study is when would BDNF be released to impact on ADBE? A number of studies have shown that BDNF is released by neurons during high-intensity stimulation [25] , [26] . Recent work using GFP-tagged BDNF in primary hippocampal cultures have suggested that the majority of BDNF that is secreted is via dendritic release, potentially feeding back to modulate presynaptic function [27] . In agreement BDNF is proposed to be released in a retrograde manner to maintain neurotransmission at the parallel fibre—Purkinje cell synapse [41] . Intense action potential firing can also lead to presynaptic BDNF release [27] . Such firing may occur in pathophysiolgical conditions such as epileptic seizure. In agreement epilepsy is associated with increased levels of BDNF [44] , which may exacerbate seizures by increasing neurotransmission via its block of ADBE. We have shown that activation of a presynaptic signalling cascade by an extracellular signalling molecule, BDNF, results in inhibition of GSK3 activity, the arrest of both dynamin Ser-774 rephosphorylation and ADBE and finally enhancement of neurotransmission during high-frequency stimulation. This suggests that different SV endocytosis modes, and ADBE in particular, may be a potential target for strategies to modify synaptic strength in either neurodegenerative conditions or disorders of neuronal excitability such as epilepsy. Materials FM2-10, tetramethyrhodamine-dextran, Lipofectamine 2000, penicillin/streptomycin, phosphate buffered salts, fetal calf serum and minimal essential medium, were obtained from Life Technologies (Paisley, UK). Synaptophysin antibody was from Synaptic Systems (Germany). The dynamin I phosphospecific Ser-774 and Ser-778 antibodies were from AbD Serotec (Cambridge, UK). The phospho-Akt Ser-473 and phospho-GSK3 β/α Ser-9/21 antibodies were from Cell Signalling (Herts, UK). Glutaraldehyde and osmium tetroxide were from Agar Scientific (Essex, UK). BDNF was from Cambridge Bioscience (Cambridge, UK). Bafilomycin A1 was from Acros Organics (Loughborough, UK). CT99021 was from Stratech Scientific (Suffolk, UK). Full-length rat dynamin Ixa was fused to the fluorescent protein mCerulean at its C terminus, with the Ser774Ala mutation generated by site-directed mutagenesis [9] . SypHy was generated by inserting the pH-sensitive green fluorescent protein, pHlourin at the second intravesicular loop of rat synaptophysin [2] . All other reagents were from Sigma (Poole, UK). Primary cell culture In all cases, animals were killed by schedule 1 procedures in accordance with UK Home Office Guidelines. Primary cultures of CGNs were prepared from the cerebella of 7-day-old Sprague–Dawley rat pups of either sex [45] . Cultures were used between 8–12 days in vitro . For all experiments, cultures were removed from culture medium into incubation medium (in mM: 170 NaCl, 3.5 KCl, 0.4 KH 2 PO 4 , 20 TES ( N -tris(hydroxy-methyl)-methyl-2-aminoethane-sulfonic acid), 5 NaHCO 3 , 5 glucose, 1.2 Na 2 SO 4 , 1.2 MgCl 2 , 1.3 CaCl 2 , pH 7.4) for 10 min before commencing experiments. Assays of protein phosphorylation status After equilibration in incubation medium (10 min), cultures were rested in incubation medium for a further 10 min in the presence or absence of compounds. Cultures were then stimulated for 1 min with 50 mM KCl (50 mM NaCl removed to maintain osmolarity) and allowed to repolarize for 10 min in incubation medium. CGNs were immediately lysed in SDS sample buffer (67 mM SDS, 2 mM EGTA, 9.3% glycerol, 12% β-mercaptoethanol, bromophenol blue, 67 mM Tris, pH 7.4) after either the 10 min rest phase (Basal), the 1 min stimulation, or after the repolarization phase. Lysate was quickly removed and boiled for subsequent analysis by SDS–PAGE and western blotting. Where indicated BDNF, LY294002 or K252a were included in the incubation medium before (10 min), during and after stimulation. All primary antibodies were used at a dilution of 1:1,000. The intensity of the signal from the phospho-dynamin, phospho-GSK3 and phospho-Akt blots was normalized against synaptophysin on the same western blot and expressed as a percentage of basal phosphorylation. The full version of all cropped western blots displayed in this manuscript can be viewed in Supplementary Figs S6–S8 . Fluorescence imaging of dextran uptake Uptake of tetramethyrhodamine-dextran (40 kDa) was monitored in the following manner. For S1 experiments, CGNs were left for 10 min in incubation medium and then stimulated with a train 800 action potentials (80 Hz 10 s) in the presence of 50 μM tetramethyrhodamine-dextran. Action potentials were delivered using a Warner Instruments field stimulation chamber (RC-21BRFS) with parallel platinum wires (6 mm apart). Cultures were stimulated with 1 ms pulses of 100 mA for all conditions. For the S2 experiments, CGNs were stimulated with 50 mM KCl for 1 min after a 10 min rest in incubation medium. Cultures were then repolarized for 10 min and then stimulated with 800 action potentials (80 Hz) in the presence of tetramethyrhodamine dextran. BDNF or LY294002 were present for 10 min before S1 stimulation and at all points thereafter where indicated. Dextran loading was determined by the number of fluorescent puncta in a defined field of view for untransfected neurons using a × 20 air objective at 550 nm excitation and >575 nm emission on a Zeiss Axio-observer D1 inverted epi-fluorescence microscope. The number of dextran puncta per field was quantified using FIJI (National Institutes of Health). The images were first thresholded using the Max-Entropy algorithm and the number of puncta (between 1–3.5 μm 2 ) counted. The average number of dextran puncta per field for each experiment (usually 10 fields of view per experiment) were averaged for the same conditions and the value for the unstimulated background was subtracted to give the corrected dextran uptake. At least four independent experiments were performed for each experimental condition. Monitoring of sypHy fluorescence CGNs were transfected with the genetic reporter sypHy [2] using lipofectamine 2000 between 4–6 days in vitro . Transfected neurons were imaged after 72 h using a × 40 oil immersion objective and 480 nm excitation and >525 nm emission on a Zeiss Axio-Observer D1 inverted epi-fluorescence microscope. After a 40 s period to establish a stable baseline, bafilomycin A1 (200 nM) was added to the imaging chamber. The sypHy response was recorded for a further 10 min (to visualize spontaneous SV-fusion events) before challenging with a train of 800 action potentials delivered at 80 Hz (to visualize evoked SV fusion). After recording for a further 3 min, incubation medium supplemented with 50 mM NH 4 Cl (NaCl removed to maintain osmolarity) was perfused into the chamber to reveal the remaining quenched sypHy fluorescence. BDNF (100 ng ml −1 ) was added coincident with bafilomycin A1 and remained present throughout the remainder of the experiment where indicated. The fluorescence readout from defined regions of interest from transfected neurons was recorded and normalized to the peak sypHy response in the presence of NH 4 Cl. The peak response during both spontaneous (after 10 min) and evoked (after 800 action potentials) was calculated as a function of the total SV pool (revealed by NH 4 Cl addition). Labelling of endocytosis pathways by HRP Cells were processed for HRP labelling as described below. For S1 experiments, cultures were stimulated for 2 min with stimulation medium (50 mM KCl) supplemented with HRP (10 mg ml −1 ) after 10 min in incubation medium. For S2 experiments CGNs were treated identically to S1 stimulated cultures (no HRP added in S1 stimulation solution) but then repolarized in incubation medium for 10 min before a second exposure to stimulation medium supplemented with HRP (10 mg ml −1 ). Cells were fixed immediately after either S1 or S2 in a 2% solution of glutaraldehyde in phosphate buffered saline for 30 min at 37 °C. After washing with 100 mM Tris (pH 7.4), cells were exposed to 0.1% diaminobenzidine and 0.2% H 2 O 2 in 100 mM Tris. On development of colour, they were washed with 100 mM Tris then stained with 1% osmium tetroxide for 30 min. After washing, they were post-stained with 2% uranyl acetate for 15 min and dehydrated using ethanol series and polypropylene oxide and embedded using Durcupan. Samples were sectioned, mounted on grids and viewed using a FEI Tecnai 12 transmission electron microscope (Oregon, USA). Where indicated, cells were incubated with BDNF (100 ng ml −1 ) for 10 min before the first KCl stimulus and at all points subsequent. Nerve terminals that contained HRP were analysed and intracellular structures that were less than 100 nm in diameter were arbitrarily designated to be SVs, whereas larger structures were designated to be endosomes. Cerebellar slice electrophysiology Sagital cerebellar slices (250 μm) were prepared from postnatal day 16–21 male Sprague–Dawley rats in ice-cold modified artificial CSF (ACSF) containing the following (in mM): 60 NaCl, 118 sucrose, 26 NaHCO 3 , 2.5 KCl, 11 glucose, 1.3 MgCl 2 and 1 NaH 2 PO 4 at pH 7.4 when bubbled with 95% O 2 , 5% CO 2 . Slices were incubated at 30 °C in standard ACSF containing (in mM) 119 NaCl, 2.5 CaCl 2 , 26 NaHCO 3 , 2.5 KCl, 11 glucose, 1.3 MgCl 2 , 1 NaH 2 PO 4 (pH 7.4 when bubbled with 95% O 2 : 5% CO 2 ) for 30 min then maintained at room temperature. Before transfer to the recording chamber slices were incubated for 1 h at room temperature in standard recording ACSF containing combinations of either BDNF (100 ng ml −1 ), LY294002 (10 μM) or CT99021 (2 μM). For control recordings, slices were also incubated for 1 h at room temperature in standard ACSF. Upon transfer to the recording chamber, slices were continuously perfused (3–5 ml min −1 at 32 °C) with the same solution in which they were incubated. Whole-cell, voltage clamp recordings were made from visually identified Purkinje neurons held at −60 mV using a Multiclamp 700B amplifier (Axon Instruments) and boroscillicate patch-pipettes (3–5 MΩ) filled with an internal recording solution containing (in mM) 130 caesium methylsulphonate, 10 CsCl, 10 HEPES, 0.1 EGTA, 10 glucose, 10 sodium phosphocreatine, 4 Mg-ATP, 0.5 Mg-GTP and 5 QX-314 (pH 7.3 with CsOH). CT99021 (2 μM) was added to the internal solution to abolish any postsynaptic effects due to GSK3 inhibition under the different treatments. Series resistances (typically <15 MΩ) were monitored throughout and experiments were excluded when this varied by >15%. Whole-cell currents were filtered at 5 kHz and digitized at 10 kHz. Constant voltage (4–12 V, 200 μs) stimuli were delivered at 40 Hz for 15 s (600 pulses). EPSC amplitudes were measured using the NeuroMatic function in IGOR Pro (WaveMetrics Inc.). The amplitudes of every 10 consecutive EPSCs were pooled then normalized to the peak amplitude of the first EPSC. Normalized EPSC amplitudes were plotted against stimulus number to assess activity-evoked run-down of synaptic currents. The stimulating electrode was placed in the molecular layer 150–250 μm from the cell body towards the pia edge. Hippocampal cell culture Primary cultures of hippocampal neurons were prepared from E17.5 mice of either sex [46] . All animals were killed by schedule 1 procedures as defined by Home Office Guidelines. Cultures were used between 14–15 days in vitro . For all experiments, cultures were removed from culture medium into hippocampal imaging medium (in mM: 119 NaCl, 2.5 KCl, 2 CaCl 2, 2 MgCl 2 , 25 HEPES, 30 glucose, 0.01 CNQX, 0.05 APV, pH 7.4) for 10 min before commencing experiments. Dextran uptake in transfected neurons For dextran uptake in transfected neurons, CGNs were transfected with DNA encoding either wild-type or S774A mutant dynamin I tagged with mCerulean using lipofectamine 2000 after 6 days in vitro and imaged after 8 days in vitro [9] . Transfected neurons were located by viewing at 430 nm excitation (emission >525 nm). Dextran uptake was quantified as the number of dextran puncta per 100 μm of transfected neurite (usually five fields of view per experiment). Neurite length was measured using the Simple Neurite Tracer algorithm in FIJI. The unstimulated background was subtracted to give the corrected dextran uptake. At least three independent experiments were performed for each experimental condition. Statistical analysis Two sample sets were compared using a Student’s t- test, whereas sample sets greater than two were compared using a one-way ANOVA. How to cite this article: Smillie, K. J. et al . Control of synaptic vesicle endocytosis by an extracellular signalling molecule. Nat. Commun. 4:2394 doi: 10.1038/ncomms3394 (2013).